Nuclear magnetic resonance spectroscopy with single spin sensitivity Nuclear magnetic resonance spectroscopy and magnetic resonance imaging at the ultimate sensitivity limit of single molecules or single nuclear spins requires fundamentally new detection strategies. The strong coupling regime, when interaction between sensor and sample spins dominates all other interactions, is one such strategy. In this regime, classically forbidden detection of completely unpolarized nuclei is allowed, going beyond statistical fluctuations in magnetization. Here we realize strong coupling between an atomic (nitrogen–vacancy) sensor and sample nuclei to perform nuclear magnetic resonance on four 29 Si spins. We exploit the field gradient created by the diamond atomic sensor, in concert with compressed sensing, to realize imaging protocols, enabling individual nuclei to be located with Angstrom precision. The achieved signal-to-noise ratio under ambient conditions allows single nuclear spin sensitivity to be achieved within seconds. Nuclear magnetic resonance (NMR) spectroscopy is an informative tool routinely used to determine the chemical makeup of macromolecules, including large proteins [1] . Yet the weak interaction strength between sample spins and inductive detectors, and low-thermal polarization, restricts the sensitivity to large ensembles ( Fig. 1a ). The resolution of imaging techniques is additionally limited by the maximum magnetic gradient that can be applied. By miniaturizing the detector to approach the sample closer, sensor-sample coupling can be increased. Recently, magnetic resonance force microscopy [2] , [3] and diamond based magnetometers [4] , [5] , [6] have been able to demonstrate NMR on nanoscale ensembles of nuclear spins, improving sensitivity by orders of magnitude compared with the best inductive readout [7] . When noise, in the form of magnetic coupling between sample nuclear spins, exceeds interaction with the sensor, the sensitivity is classically restricted to measurements of statistical fluctuations in sample magnetization [8] ( Fig. 1b ). However, when coupling between the sensor and measured nuclei dominates over decoherence (strong coupling regime shown in Fig. 1c ), individual nuclei may be detected regardless of their polarization. Here we realize such strong coupling by bringing a single electronic spin sensor close to (~2 nm) weakly interacting 29 Si nuclei in a silica layer. Furthermore, strong coupling enables the dipolar field of the atomic sensor to be used as field gradient for magnetic resonance imaging, allowing the positions of four single nuclear spins to be imaged. The ambient experimental methods we demonstrate are an important step towards non-destructive imaging of single biomolecules under physiological conditions, and determining nanoscale structure and composition without ensemble averaging. 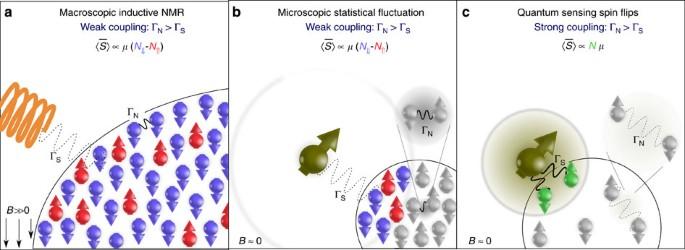Figure 1: Classical and quantum NMR detection regimes. (a) Inductive NMR: Interaction between the sensor and individual nuclear spins (ΓS) is much weaker than interaction between nuclei (ΓN). For large spin ensembles (≳1012nuclear spins) the time-averaged signal,is proportional to the sample polarization (multiplied by the spin magnetic moment,μ). In the high temperature limit, sample magnetization is, whereNis the number of spins,Bis the external magnetic field,Tis the temperature andkBis the Boltzmann constant. (b) Nanoscale NMR: For detection of small ensembles (~104nuclear spins) with a weakly coupled sensor,is still proportional to the sample magnetization. Now statistical fluctuations may exceed thermal polarization, so sample magnetization is given by. (c) Quantum NMR: Detection of individual or few nuclei may occur when interaction of each nuclear spin with the sensor (ΓS) is stronger than the coupling to the surrounding bath (ΓN). In this strong coupling regime, the magnetic field of individual spins is measured rather than sample magnetization. The detected signal,, is then proportional toNμregardless of whether the nuclei have a net polarization. Figure 1: Classical and quantum NMR detection regimes. ( a ) Inductive NMR: Interaction between the sensor and individual nuclear spins (Γ S ) is much weaker than interaction between nuclei (Γ N ). For large spin ensembles ( ≳ 10 12 nuclear spins) the time-averaged signal, is proportional to the sample polarization (multiplied by the spin magnetic moment, μ ). In the high temperature limit, sample magnetization is , where N is the number of spins, B is the external magnetic field, T is the temperature and k B is the Boltzmann constant. ( b ) Nanoscale NMR: For detection of small ensembles (~10 4 nuclear spins) with a weakly coupled sensor, is still proportional to the sample magnetization. Now statistical fluctuations may exceed thermal polarization, so sample magnetization is given by . ( c ) Quantum NMR: Detection of individual or few nuclei may occur when interaction of each nuclear spin with the sensor (Γ S ) is stronger than the coupling to the surrounding bath (Γ N ). In this strong coupling regime, the magnetic field of individual spins is measured rather than sample magnetization. The detected signal, , is then proportional to Nμ regardless of whether the nuclei have a net polarization. Full size image The nitrogen–vacancy (NV) defect in diamond is a remarkable magnetic sensor. Optically detected magnetic resonance enables the NV electronic spin to be interrogated by fluorescence microscopy [9] , and dipolar interaction with nearby spins—either in the diamond [10] , [11] , [12] or near the surface [13] , [14] , [15] , [16] , [17] , [18] , [19] , [20] allows spin spectroscopy to be performed. Other applications include nanoscale magnetic field measurements [21] , [22] , bioimaging under ambient conditions [16] , [23] , [24] , [25] and quantum information processing [26] , [27] , [28] , [29] , [30] . In the following, we focus on the possibility to achieve direct flip-flops with unpolarized nuclear spins, that is, independent of the initial state of the nuclear spin. The sensitivity of this protocol depends critically on the stand-off distance between the NV sensor and target spins, not only because the interaction strength scales inversely with the third power of the separation distance, but also because the signal characteristics change drastically when the interaction strength between NV and nuclear spins exceeds the coupling between target nuclei. In this strong coupling regime, all nuclear spins directly impart phase accumulation on the NV sensor before spin flips between nuclei occurs, which act to randomize the phase accumulation. The result is a enhancement in the signal for detection of N nuclei when compared with the classical case (see Fig. 1b,c ), without requiring sample hyperpolarization [31] . The sensitivity we achieve allows in principle a single, unpolarized nuclear spin to be detected within 10 s. Sensor creation and sensing protocol A schematic of the experiment is shown in Fig. 2a . NV defects were created by implantation of 2.5 keV N + ions into an unpolished diamond surface. Isotopically purified diamond ( 13 C concentration <10 p.p.m.) was used to avoid nuclear spin noise from intrinsic 13 C nuclei. Shallow NV centres of 2–3 nm depth ( Supplementary Table 1 ) were identified with sub-nanometre precision by placing a standard sample on the surface (see Methods, Supplementary Notes 1–3 , Supplementary Figs 1–6 ). Amorphous silica (SiO 2 ) was then deposited on the diamond surface. Silica was chosen since it has a low abundance of nuclear spins, 29 Si being the most common spin isotope with 4.67% atomic abundance. Use of a dilute spin sample allows the strong coupling regime to be attained, since 29 Si nuclear spins at the surface experience a dipolar magnetic field from nearby NV centres, which is stronger than the internuclear coupling, exceeding even the coupling between 29 Si dimers ( Fig. 2b ). In addition, the low density of 1 spin nm −3 means on average very few spins are present in the sensing volume ( Supplementary Note 4 , Supplementary Figs 7 and 8 ). 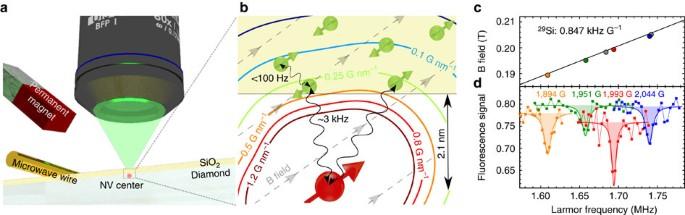Figure 2: NMR of29Si nuclei with a strongly coupled sensor. (a) Schematic of the experimental setup. Dilute, unpolarized nuclear spins in a silica layer interact with an electronic spin in a (100)-surface diamond, which is readout with optical microscopy. (b) Schematic of strong coupling regime. A shallow NV centre in diamond (2 nm from the surface) couples to nearby29Si nuclei in a silica layer, due to hyperfine interaction. The contour lines show the strength of the effective magnetic gradient experienced by the nuclear spins. (c) Measured29Si NMR signal as a function of applied magnetic field, using the XY8-Kdecoupling sequence. The detected signal has a slope of 0.847(1) kHz G−1in agreement with the gyromagnetic ratio for29Si (solid line). The systematic shift of the detected frequency is due to the finite temporal length of decoupling pulses on the NV sensor. (d) Measured echo dip for NV centres at different magnetic fields. The signal dependence on the decoupling pulse number can be seen by comparing the data sets at 1,894, 1,951 and 2,044 Gauss (64 pulse acquisition), to the data set at 1,993 Gauss (128 pulse acquisition). Higher-order pulses produce a narrower signal with a stronger dip, up to the decoherence time. Fluorescence contrast has been normalized to the level corresponding to a complete NV spin flip. Measurements at 1,894, 1,993 Gauss were performed on NV-6 with a nominal depth of 2.1 nm, measurements at 1,951, 2,044 Gauss were performed on NV-7 with a depth of 2.3 nm. Figure 2: NMR of 29 Si nuclei with a strongly coupled sensor. ( a ) Schematic of the experimental setup. Dilute, unpolarized nuclear spins in a silica layer interact with an electronic spin in a (100)-surface diamond, which is readout with optical microscopy. ( b ) Schematic of strong coupling regime. A shallow NV centre in diamond (2 nm from the surface) couples to nearby 29 Si nuclei in a silica layer, due to hyperfine interaction. The contour lines show the strength of the effective magnetic gradient experienced by the nuclear spins. ( c ) Measured 29 Si NMR signal as a function of applied magnetic field, using the XY8- K decoupling sequence. The detected signal has a slope of 0.847(1) kHz G −1 in agreement with the gyromagnetic ratio for 29 Si (solid line). The systematic shift of the detected frequency is due to the finite temporal length of decoupling pulses on the NV sensor. ( d ) Measured echo dip for NV centres at different magnetic fields. The signal dependence on the decoupling pulse number can be seen by comparing the data sets at 1,894, 1,951 and 2,044 Gauss (64 pulse acquisition), to the data set at 1,993 Gauss (128 pulse acquisition). Higher-order pulses produce a narrower signal with a stronger dip, up to the decoherence time. Fluorescence contrast has been normalized to the level corresponding to a complete NV spin flip. Measurements at 1,894, 1,993 Gauss were performed on NV-6 with a nominal depth of 2.1 nm, measurements at 1,951, 2,044 Gauss were performed on NV-7 with a depth of 2.3 nm. Full size image To detect hyperfine interaction between the NV defect and N unpolarized nuclei, we bring the NV spin into resonance with nuclear spins, and then read the phase acquired by the NV due to interaction with the nuclei. Nuclear evolution is governed by the Hamiltonian: where S i and I i are the NV electron and 29 Si nuclear spin operators respectively, ω L is the Larmor frequency, and α , β are the parallel and perpendicular components of the hyperfine coupling (see Supplementary Note 5 ). The hyperfine interaction (second term of Eq. 1) is zero for NV in the | m s =0› state of the magnetic ground-state triplet, whereas for the NV | m s = −1› state, each nuclear spin rotates about an axis set by the vector sum of the external magnetic field and the positional-dependent hyperfine field. By repeated adjustments of the NV spin state in synchrony with nuclear evolution, the nuclear trajectory can be tailored to allow a complete flip, (in concert with an NV flop)—in effect, amplifying the conditional interaction. The rate of this rotation is given by the perpendicular component ( β ) of the hyperfine interaction, and we emphasize that rotation occurs independently of whether the nucleus was initially spin up or spin down. For several nuclei each with individual coupling rates, the dynamics of the sensor become complex; however, in the short time limit investigated here, the overall signal closely approximates a linear sum of individual contributions (see Supplementary Note 6 and Supplementary Figs 9–12 ). The particular pulse sequence we used to adjust the NV spin state in time with nuclear evolution was the XY8- K pulse sequence, as it is robust against pulse errors [32] . The optimum timing of pulses on the NV spin to produce a spin flip is given by where m =1, 3, 5 ..., arises due to the periodicity of the rotation—referred to as the order of the dip [10] , and f n is the frequency of each nuclear spin, which may be shifted from the bare Larmor frequency by hyperfine interaction with the NV spin. Dynamical decoupling also protects the NV from unwanted spin noise, in particular at high fields where the decoupling pulses are dense, and for this reason, we operated at magnetic fields of ~0.2 T. NMR spectroscopy of few nuclear spins In Fig. 2c,d , we plot the measured XY8 spin echo for NV spins below the silica interface, which shows a clear dip near the 29 Si Larmor frequency, due to the relative phase acquired by the NV. Analysis of the signal strength gives agreement for interaction with six to eight nuclear spins, where we have taken into account the depth of the NV centres and the expected 29 Si density. We have verified with the parameters in our experiments ( ω L ≫ α n , β n ), that the dependence of the signal on the 29 Si nuclear spin polarization is negligible, thus demonstrating a new detection regime of NMR (more details are available in Supplementary Notes 4,5 and Supplementary Fig. 9 ). We are also able to estimate the coupling strength between NV and nuclei from the signal contrast over the measurement time. The 8% contrast we obtain over the interaction time (19 μs) gives an average coupling strength to individual nuclei on the order of 3 kHz, consistent with the perpendicular component of the hyperfine interaction for a separation between NV electron spin and 29 Si nuclear spins of 2 nm. Magnetic resonance imaging of individual nuclear spins To resolve the hyperfine couplings of individual 29 Si nuclei, we increased the number of decoupling pulses, thereby improving the spectral resolution. For a classical spin bath where a large number of equivalent spins interact weakly with the NV centre [4] , [5] , the echo dip is centred at the nuclear Larmor frequency, and its width, Δ ω scales with the sensitivity function of the echo, Δ ω /2 π ≈1/ Kτ , where K is the total number of pulses. However, in the case of strong interaction between nuclei and electron spin sensor, individual nuclei become detuned and the width of the echo dip is given by the inhomogeneous broadening resulting from the field gradient created by the electron spin [10] , [11] , [12] . Here we use the 0.05 mT nm −1 magnetic gradient at separations of 2 nm between the atomic scale NV sensor and silicon spins, as a unique opportunity for nanoscale imaging. Under higher-order decoupling, inhomogeneous broadening of the NMR signal becomes apparent ( Fig. 3a ), but broad-band magnetic noise prevented observation of full electron-nuclear flip-flops and thus fully resolved lines. We were nevertheless able to gain deeper insight into the location and detuning of individual nuclear spins by employing advanced methods from signal processing. Indeed, the frequencies of individual nuclei while not being immediately resolvable can be extracted using the superresolution properties of basis pursuit de-noising [33] (BPDN, see Methods, Supplementary Notes 7 and 8 , Supplementary Figs 13–16 ). 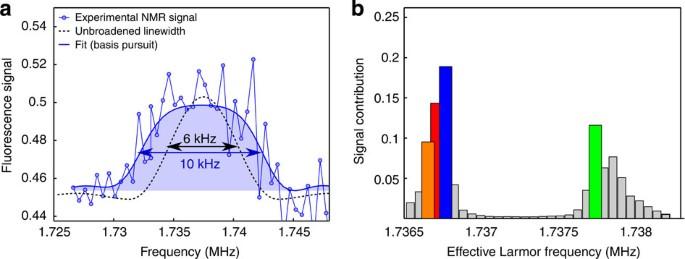Figure 3: NV gradient separation of individual29Si nuclei. (a) Under high-order decoupling (XY8-512 pulse sequence), inhomogeneous broadening of the29Si NMR line due to the NV magnetic gradient can be observed. The expected line width of the XY8-512 sequence for weakly interacting nuclear spins is shown as the black dotted line with a FWHM of 6 kHz. The blue solid line is the best fit to the data using basis pursuit (seeSupplementary Note 7for technical details) showing an additional broadening of 4 kHz. (b) Using BPDN, we calculate the Larmor frequency and relative contribution of 50 nuclear spins comprising the total signal (see Methods). These are plotted individually, with the four strongest highlighted, which contribute to more than 50% of the signal. Figure 3b shows the obtained spectral decomposition of the contributing nuclear spins and their hyperfine coupling parameters, suggesting that four nuclei account for more than 50% of the signal ( Supplementary Fig. 15 ), which is of comparable size to many chemical functional groups and below the size of a small amino acid. Figure 3: NV gradient separation of individual 29 Si nuclei. ( a ) Under high-order decoupling (XY8-512 pulse sequence), inhomogeneous broadening of the 29 Si NMR line due to the NV magnetic gradient can be observed. The expected line width of the XY8-512 sequence for weakly interacting nuclear spins is shown as the black dotted line with a FWHM of 6 kHz. The blue solid line is the best fit to the data using basis pursuit (see Supplementary Note 7 for technical details) showing an additional broadening of 4 kHz. ( b ) Using BPDN, we calculate the Larmor frequency and relative contribution of 50 nuclear spins comprising the total signal (see Methods). These are plotted individually, with the four strongest highlighted, which contribute to more than 50% of the signal. Full size image To demonstrate how structural information and imaging may be obtained, we plot the best fit locations of silicon nuclei as recovered from BPDN ( Fig. 4a ). The two-component ( α , β ) anisotropy of the hyperfine interaction allows assignment of a unique location for each nuclear spin up to one degree of circular symmetry, with respect to the NV axis. Despite the extra degree of freedom, we are still able to estimate the location of two nuclei with an uncertainty below 0.2 nanometres ( Supplementary Note 9 , Supplementary Fig. 17 ). Techniques which break the circular symmetry ( Supplementary Note 10 ) and longer data acquisition times can be used to reduce the spatial resolution below one Angstrom. 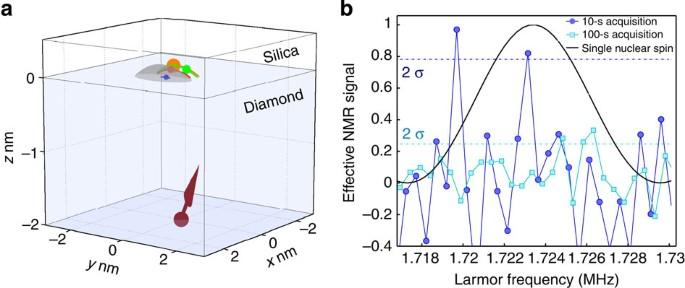Figure 4: Imaging of nuclear positions and single spin sensitivity. (a) The best fit locations of the four strongest contributing29Si nuclei as obtained from basis pursuit are shown as the coloured arcs (colour corresponds withFig. 3b). A representative position of each spin is denoted with a filled ball, and the positional uncertainty in thexandzdirections is given by the size of the ball. Maximal uncertainties from BPDN are Δx=±0.2 nm, Δz=±0.1 nm. The circular symmetry of the field pattern greatly increases the uncertainty around the azimuthal angle, here it is limited by intersection with the diamond surface; as a result, the resolution inyis 0.1 nm for the nearest spin and increases to 0.5 nm for the furthest spin (seeSupplementary Note 9). The surface of the hyperfine pattern with a strength equal to the signal plotted in (b) is shown in grey. (b) Expected NMR signal for the case of a single29Si nuclear spin on the surface of the 0.5 nm3volume shown in (a). The signal exceeds the shot noise limit by more than two s.d. values for a 9.7 s acquisition per time point (dark circles). Figure 4: Imaging of nuclear positions and single spin sensitivity. ( a ) The best fit locations of the four strongest contributing 29 Si nuclei as obtained from basis pursuit are shown as the coloured arcs (colour corresponds with Fig. 3b ). A representative position of each spin is denoted with a filled ball, and the positional uncertainty in the x and z directions is given by the size of the ball. Maximal uncertainties from BPDN are Δ x =±0.2 nm, Δ z =±0.1 nm. The circular symmetry of the field pattern greatly increases the uncertainty around the azimuthal angle, here it is limited by intersection with the diamond surface; as a result, the resolution in y is 0.1 nm for the nearest spin and increases to 0.5 nm for the furthest spin (see Supplementary Note 9 ). The surface of the hyperfine pattern with a strength equal to the signal plotted in ( b ) is shown in grey. ( b ) Expected NMR signal for the case of a single 29 Si nuclear spin on the surface of the 0.5 nm 3 volume shown in ( a ). The signal exceeds the shot noise limit by more than two s.d. values for a 9.7 s acquisition per time point (dark circles). Full size image Single nuclear spin sensitivity The signal-to-noise ratio of the experiments presented here reaches the ultimate sensitivity limit of NMR spectroscopy ( Fig. 4b ). We show that for a single point measurement time of 10 s, the signal from a single nuclear spin exceeds shot noise by more than two s.d. values. With a sensing volume on the order of a cubic nanometre and single spin sensitivity, the direct discrimination of single molecules based on differences of one atom at a functional site appears feasible. As further confirmation of detection in the strong coupling regime, we note the scaling of the signal with distance from diamond surface r is also stronger than the classical case, closely following r −3 behaviour ( Supplementary Note 6 ). The results presented in this paper show that by operating in the strong coupling regime, the sensitivity of NMR and imaging can be extended to single nuclear spins. The technique can be applied to perform two-dimensional NMR [34] on single biomolecules with spatial resolution well below the size of a protein and thus allow for label-free detection. Further improvements in decoupling techniques will allow a spectral resolution limited by the electron spin relaxation time [35] (~100 Hz for NVs measured here). Although the strong coupling regime reported in this paper allows for polarization-independent NMR, the possibility to transfer NV polarization to nearby nuclei [36] , [37] , [38] will allow for investigations of internuclear couplings and nuclear Overhauser effect. Nuclear decoupling techniques will also allow strong coupling to be achieved in dense spin samples, providing a signal independent of nuclear polarization [39] , [40] . In addition, as demonstrated here, benefits can be derived from the use of signal processing methods to extract more detailed information about spins contributing to the signal and can also allow for a significant reduction in the number of data points required [41] . Direct manipulation of nuclear spins using radiofrequency fields may be utilized as a high resolution spectroscopy tool for detection of chemical shifts, giving information on the three dimensional structure of molecules [5] , [42] . Alternatively, electron spin labels providing pseudocontact chemical shifts [43] may be employed to enable direct resolution of individual nuclei in single molecules. Calibration of NV depth and sensing volume To identify shallow NV centres, we measured the nuclear magnetic signal at the Larmor frequency of 1 H using the XY8- K dynamical decoupling sequence. Initial characterization was performed with a dense nuclear spin sample—immersion oil (Fluka Analytical 10976). The signal remained in the weak coupling regime; therefore, we use a classical treatment [4] . First, we measure the magnetic field fluctuation ‹Δ B 2 ›, from protons in the oil by integrating the power spectral density S ( ω ), see Supplementary Fig. 4 : For NV-6, plotted in Fig. 2 , we obtain , further details can be found in Supplementary Note 3 . If we assume the protons to be homogeneously distributed with a density ρ on the diamond surface in a layer of thickness h , we obtain the magnetic field sensed by an NV centre in a depth r below the diamond surface by [19] : where μ H =1.41 × 10 −26 J · T −1 is the nuclear magneton of hydrogen and μ 0 the vacuum permeability. For a proton density of 50 nm −3 , and a sample thickness exceeding 10 nm, the measured magnetic field leads to a depth estimate of 2.1 nm, with an error dominated by uncertainty in the oil density ( Supplementary Fig. 5 ). To determine the sensing volume, we analysed the signal as a function of number of nuclear spins, showing that 390–400 nuclei make the most significant contribution to the signal, corresponding to a volume of 8 nm 3 above the diamond surface (more details in Supplementary Note 3 and Supplementary Fig. 6 ). Deposition of amorphous silica on diamond surface After identification of shallow NV centres, diamonds were cleaned in a 1:1:1 admixture of three acids (H 2 SO 4 :HClO 4 :HNO 3 ) at 180 °C for several hours. After cleaning, the diamonds were transferred to chromatography grade water before ~10 μl of a 1:1 solution of (tetraethyl orthosilicate:ethanol) was dropped onto the surface. We also observed comparable results when depositing undiluted tetraethyl orthosilicate onto a diamond surface directly taken from water. Diamond substrates were then placed onto a hotplate at 120 °C for 10 min. Basis pursuit analysis BPDN determines signal representations from overcomplete dictionaries of signal forms by convex optimization [33] . The total signal, χ ( τ ) we observe, arises from 29 Si nuclei and background noise ( Supplementary Fig. 10 ), namely χ ( τ )= χ Si ( τ )+ χ bg ( τ ), with the total contribution from 29 Si nuclei, χ Si ( τ ) being summed over all N individual nuclei, . To perform this analysis, we assume that the contribution of individual 29 Si takes the form of a normalized filter function: which is based on the assumption that each individual 29 Si generates a magnetic field with a delta (effective Larmor) frequency ω n . An exact numerical simulation using the full Hamiltonian suggests that the shape of the above basis function agrees very well with the shape of the echo decay caused by a single 29 Si with a typical distance of 2–3 nm to the NV centre. The experimental data provide us with a series of function values for the echo decay C exp ( τ ). The task that BPDN solves is to reproduce the observed signal to a desired precision using a superposition of the smallest number of dictionary elements (that is, 29 Si nuclear spins). That is we solve the optimization problem where b j ≥0 quantifies the contribution of each basis function to the total signal and can be identified with perpendicular component of the hyperfine coupling by a scaling factor, b M is the maximum value b j may take, given an NV depth of 2 nm. The value of λ determines how well the fitting data should agree with the experiment data, and J is the number of basis functions. We chose J =30, meaning we take into account 30 spins to describe the signal. From the silica density, this gives a contributing volume of ~25–30 nm 3 much greater than the sensing volume, and beyond this distance, the strong coupling regime no longer holds. Using BPDN, we are able to reproduce the experimental data with very good agreement. For a smaller value of λ , the solution becomes close to the exact basis pursuit, and the fitting shows better agreement with the experiment (see Supplementary Fig. 14 and details in Supplementary Note 7 ). The estimation of the number of 29 Si that produce the observed signal is robust when varying the parameter λ in BPDN as long as the fitting is above a certain confidence level, see Supplementary Note 7 . We have verified the validity of the optimal values of b n and ω n obtained: the amplitudes b n are consistent with a distance to the NV centre of around 2 nm and the distribution of ω n that make largest contribution are within a few kHz. How to cite this article : Müller, C. et al. Nuclear magnetic resonance spectroscopy with single spin sensitivity. Nat. Commun. 5:4703 doi: 10.1038/ncomms5703 (2014).